Glycolytic genes are targets of the nuclear receptor Ad4BP/SF-1 Genetic deficiencies in transcription factors can lead to the loss of certain types of cells and tissue. The steroidogenic tissue-specific nuclear receptor Ad4BP/SF-1 (NR5A1) is one such gene, because mice in which this gene is disrupted fail to develop the adrenal gland and gonads. However, the specific role of Ad4BP/SF-1 in these biological events remains unclear. Here we use chromatin immunoprecipitation sequencing to show that nearly all genes in the glycolytic pathway are regulated by Ad4BP/SF-1. Suppression of Ad4BP/SF-1 by small interfering RNA reduces production of the energy carriers ATP and nicotinamide adenine dinucleotide phosphate, as well as lowers expression of genes involved in glucose metabolism. Together, these observations may explain tissue dysgenesis as a result of Ad4BP/SF-1 gene disruption in vivo . Considering the function of estrogen-related receptor α, the present study raises the possibility that certain types of nuclear receptors regulate sets of genes involved in metabolic pathways to generate energy carriers. The production of important coenzymes for energy potential and reducing power, for example, ATP and nicotinamide adenine dinucleotide phosphate (NADPH), is mediated by nutrient catabolism. Glucose, the representative nutrient, is catabolized through the glycolytic pathway, and subsequently by the tricarboxylic acid (TCA) cycle and oxidative phosphorylation. This sequential process ultimately produces ATP, which thereafter serves as the energy source for many metabolic processes. Alternatively, glucose is catabolized through the pentose phosphate pathway (PPP) to synthesize ribose-5-phosphate and NADPH. The former is essential for nucleic acid synthesis, whereas the latter is required for the reductive biosynthesis of fatty acids, cholesterol and steroid hormones, among others. Together, these two glucose catabolic pathways are necessary for a variety of cellular processes. Ad4BP/SF-1 (NR5A1), a member of the nuclear receptor superfamily, is expressed specifically in the steroidogenic adrenal cortex and gonads [1] , [2] , [3] , [4] , [5] . This protein was originally identified as a transcription factor that regulated the steroidogenic CYP11A1 and CYP11B1 genes [6] ; subsequent studies eventually demonstrated that all steroidogenic genes are targets of Ad4BP/SF-1 (refs 7 , 8 ). To date, a collective body of work has established that Ad4BP/SF-1 controls steroid hormone synthesis through the transcriptional regulation of all steroidogenic genes. In addition to steroidogenic regulation, Ad4BP/SF-1 has a crucial role in steroidogenic tissue development as revealed by mice bearing targeted deletions in the gene. Namely, those animals lacked steroidogenic tissues, such as adrenal glands and gonads [9] , [10] , [11] , [12] . By contrast, the overexpression of Ad4BP/SF-1 induced enlargement/ectopic formation and tumorigenesis of the adrenal cortex [13] , [14] , [15] , [16] . Taken together, these studies strongly suggested that Ad4BP/SF-1 is involved in the regulation of cellular proliferation and maintenance. However, it is unlikely that Ad4BP/SF-1 controls cellular proliferation and maintenance through steroidogenic gene regulation. Here we investigate how Ad4BP/SF-1 regulates such cellular events. The results reveal that Ad4BP/SF-1 is strongly implicated in glucose metabolism by governing the coordinated regulation of genes within a glycolytic pathway. Glycolytic gene expression affected by Ad4BP/SF-1 knockdown Cultured adrenocortical Y-1 cells [17] , which express Ad4BP/SF-1, were used to examine whether cellular proliferation would be affected by knockdown with small interfering RNA (siRNA; mixture of three siRNAs) targeting Ad4BP/SF-1 (si Ad4BP/SF-1 ) or control siRNA (siControl). Treatment with si Ad4BP/SF-1 reduced the expression of Ad4BP/SF-1 mRNA and protein by approximately 80% ( Fig. 1a,b ). Consistent with previous reports [18] , [19] , [20] , [21] , the treated cells were decreased in number, probably due to decreased proliferation ( Fig. 1c,d ). To examine which genes were regulated by Ad4BP/SF-1, we performed deep sequencing of RNA prepared from Y-1 cells treated with these siRNAs. We expected that genes necessary for cell proliferation would be contained in the genes whose expression was decreased by si Ad4BP/SF-1 treatment. Although gene expression was mostly unaffected by the treatment, the expression of 1.47% (243) of genes was decreased by <50%, and the expression of 1.96% (324) of genes was increased by >200% in the si Ad4BP/SF-1 -treated cells ( Fig. 2a ; Supplementary Fig. 1 ; Supplementary Data 1 and 2 ). Although it remains to be examined whether these genes were regulated directly by Ad4BP/SF-1, a chromatin immunoprecipitation (ChIP)-seq study described below indicated that ChIP-peaks for Ad4BP/SF-1 are localized within 10 kb of a transcription start or stop site in 21.0% of the downregulated and 9.2% of the upregulated genes. Given that these genes are direct targets of Ad4BP/SF-1, it would be interesting to delineate the mechanisms through which the opposite functions, either transcriptional activation or suppression, are mediated. Sequences surrounding Ad4BP/SF-1-binding site would contribute to alternative selection from the opposite functions of Ad4BP/SF-1. 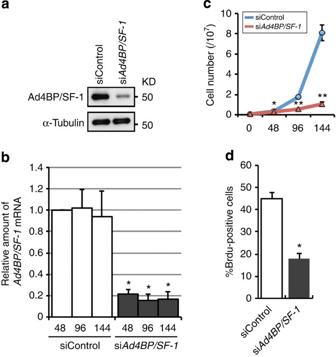Figure 1:Ad4BP/SF-1knockdown leads to decreased proliferation in Y-1 cells. (a) Whole-cell lysates prepared from Y-1 cells treated for 96 h with siControl or siAd4BP/SF-1were subjected to immunoblotting to examine the expression levels of Ad4BP/SF-1. A pool of small interfering RNA (siRNAs; see Methods) was used. α-Tubulin was used as a control. Full blot images are shown inSupplementary Fig. 21. (b) Y-1 cells were treated with siControl (white) or siAd4BP/SF-1(black) for 48, 96 or 144 h. Total RNAs prepared from the cells were subjected to quantitative reverse transcription–PCR to assessAd4BP/SF-1expression. Average values and SDs are indicated (b–d). The average value for the siControl-treated cells (48 h) was normalized to 1.0. *P<0.005.n=3. (c) The number of Y-1 cells was determined at 48, 96 and 144 h after treatment with siAd4BP/SF-1(red) or siControl (blue). *P<0.025, **P<0.005.n=3. (d) Cell proliferation was examined by 5-bromodeoxyuridine (BrdU) incorporation in siAd4BP/SF-1-(black) and siControl- (white) treated Y-1 cells. The cells were treated with the siRNA for 96 h, cultured with 100 μM BrdU for 3 h, and then subjected to immunohistochemical analysis with antibodies against BrdU to detect proliferating cells. The percentages of BrdU-positive cells are indicated. *P<0.005.n=3. The statistical significances were examined using a two-tailed Student’st-test (b–d). Figure 1: Ad4BP/SF-1 knockdown leads to decreased proliferation in Y-1 cells. ( a ) Whole-cell lysates prepared from Y-1 cells treated for 96 h with siControl or si Ad4BP/SF-1 were subjected to immunoblotting to examine the expression levels of Ad4BP/SF-1. A pool of small interfering RNA (siRNAs; see Methods) was used. α-Tubulin was used as a control. Full blot images are shown in Supplementary Fig. 21 . ( b ) Y-1 cells were treated with siControl (white) or si Ad4BP/SF-1 (black) for 48, 96 or 144 h. Total RNAs prepared from the cells were subjected to quantitative reverse transcription–PCR to assess Ad4BP/SF-1 expression. Average values and SDs are indicated ( b – d ). The average value for the siControl-treated cells (48 h) was normalized to 1.0. * P <0.005. n =3. ( c ) The number of Y-1 cells was determined at 48, 96 and 144 h after treatment with si Ad4BP/SF-1 (red) or siControl (blue). * P <0.025, ** P <0.005. n =3. ( d ) Cell proliferation was examined by 5-bromodeoxyuridine (BrdU) incorporation in si Ad4BP/SF-1- (black) and siControl- (white) treated Y-1 cells. The cells were treated with the siRNA for 96 h, cultured with 100 μM BrdU for 3 h, and then subjected to immunohistochemical analysis with antibodies against BrdU to detect proliferating cells. The percentages of BrdU-positive cells are indicated. * P <0.005. n =3. The statistical significances were examined using a two-tailed Student’s t -test ( b – d ). 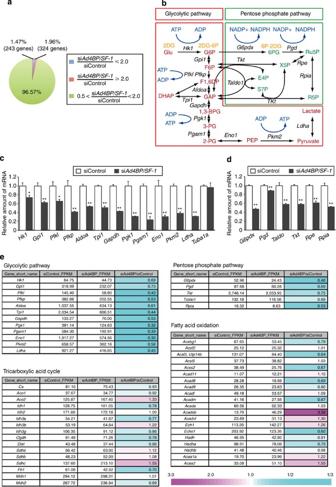Figure 2: Glycolytic gene expression is affected byAd4BP/SF-1knockdown. (a) The expression levels of 1.47% (243) genes were decreased to less than 50% of control values (blue) by siAd4BP/SF-1treatment, whereas 1.96% (324) genes increased expression levels by more than 200% (red). Meanwhile, the expression levels of the majority of genes (96.57%) expressed in Y-1 cells were not affected by siAd4BP/SF-1treatment (green). (b) Intermediate metabolites and genes involved in the glycolytic and pentose phosphate pathway (PPP) are shown. Reactions coupled with nicotinamide adenine dinucleotide phosphate (NADPH) synthesis and ATP consumption and synthesis are indicated. Metabolites derived from 2-deoxyglucose (2DG) are shown (orange; seeFig. 7). Abbreviations are defined inSupplementary Table 3. (c,d) The expression of the glycolytic (c) and PPP genes (d) was compared between cells treated with siAd4BP/SF-1(black bar) and siControl (white bar) using quantitative reverse transcription–PCR. Average values and SDs are indicated (c,d). The average values for the siControl-treated cells were normalized to 1.0. *P<0.025, **P<0.005.n=3. The statistical significances were examined using a two-tailed Student’st-test (c,d). (e) Expression of genes constituting metabolic pathways (glycolysis, tricarboxylic acid cycle, PPP and fatty acid oxidation) affected by siAd4BP/SF-1treatment. Each table shows gene names, expression levels in the cells treated with siControl, expression levels in the cells treated with siAd4BP/SF-1and ratios of the expressions (siAd4BP/SF-1/siControl), as indicated at the top. Magenta and turquoise indicate up- and downregulated expression, respectively. Gradient of the colour represents levels of changes in gene expression; darker colours indicate larger changes. FPKM, fragments per kilobase of transcript per million mapped fragment. Full size image Figure 2: Glycolytic gene expression is affected by Ad4BP/SF-1 knockdown. ( a ) The expression levels of 1.47% (243) genes were decreased to less than 50% of control values (blue) by si Ad4BP/SF-1 treatment, whereas 1.96% (324) genes increased expression levels by more than 200% (red). Meanwhile, the expression levels of the majority of genes (96.57%) expressed in Y-1 cells were not affected by si Ad4BP/SF-1 treatment (green). ( b ) Intermediate metabolites and genes involved in the glycolytic and pentose phosphate pathway (PPP) are shown. Reactions coupled with nicotinamide adenine dinucleotide phosphate (NADPH) synthesis and ATP consumption and synthesis are indicated. Metabolites derived from 2-deoxyglucose (2DG) are shown (orange; see Fig. 7 ). 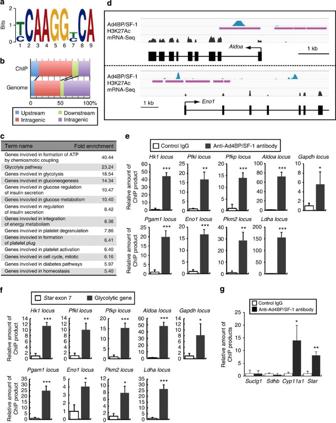Figure 3: Binding of Ad4BP/SF-1 to glycolytic gene loci. (a) The nucleotide sequence extracted from the chromatin immunoprecipitation (ChIP)-peaks of Ad4BP/SF-1 is indicated. (b) The ChIP-peaks were classified into four groups according to their relative positions to the nearest genes. (c) Genes in which the ChIP-peaks for Ad4BP/SF-1 were localized within regions ranging from 10 kb upstream to 10 kb downstream from the transcription start site were subjected to pathway analysis27,28. Term name and fold enrichment are indicated. (d) The ChIP-peaks are shown for the glycolytic genes,AldoaandEno1. Other genes are shown inSupplementary Figs 6–9. Blue histograms and purple bars indicate the ChIP-peaks of Ad4BP/SF-1 and H3K27Ac regions, respectively. Black boxes indicate exons. (e) Chromatin immunoprecipitates recovered with an anti-Ad4BP/SF-1 antibody (black) or control IgG (white) were subjected to quantitative PCR (qPCR) to detect glycolytic genes. Average values and SDs of relative amounts of the ChIP-qPCR products are shown (e–g). The average values of the control products were normalized to 1.0. *P<0.05, **P<0.01, ***P<0.005.n=3. (f) Chromatin immunoprecipitates recovered with an anti-Ad4BP/SF-1 antibody were subjected to qPCR analysis for the glycolytic genes (black bars) and exon 7 of theStargene, a negative control for Ad4BP/SF-1 accumulation (white bars). The average values for theStargene locus were normalized to 1.0. *P<0.05. **P<0.01. ***P<0.005.n=3. (g) ChIP-qPCR for genes involved in tricarboxylic acid cycle (Suclg1andSdhb) and steroidogenesis (Cyp11a1andStar). *P<0.05, **P<0.01.n=3. The statistical significances were examined using a two-tailed Student’st-test (e–g). Abbreviations are defined in Supplementary Table 3 . ( c , d ) The expression of the glycolytic ( c ) and PPP genes ( d ) was compared between cells treated with si Ad4BP/SF-1 (black bar) and siControl (white bar) using quantitative reverse transcription–PCR. Average values and SDs are indicated ( c , d ). The average values for the siControl-treated cells were normalized to 1.0. * P <0.025, ** P <0.005. n =3. The statistical significances were examined using a two-tailed Student’s t -test ( c , d ). ( e ) Expression of genes constituting metabolic pathways (glycolysis, tricarboxylic acid cycle, PPP and fatty acid oxidation) affected by si Ad4BP/SF-1 treatment. Each table shows gene names, expression levels in the cells treated with siControl, expression levels in the cells treated with si Ad4BP/SF-1 and ratios of the expressions (si Ad4BP/SF-1 /siControl), as indicated at the top. Magenta and turquoise indicate up- and downregulated expression, respectively. Gradient of the colour represents levels of changes in gene expression; darker colours indicate larger changes. FPKM, fragments per kilobase of transcript per million mapped fragment. Full size image Gene ontology analysis [22] of the downregulated genes raised the possibility that Ad4BP/SF-1 was involved in a variety of metabolic processes ( Supplementary Table 1 ). Interestingly, many of the processes included the glycolytic pathway. In fact, in addition to the steroidogenic genes, Cyp11a1 and Star , which had been previously established as targets of Ad4BP/SF-1, the expression of all glycolytic genes ( Hk1, Gpi1, Pfkl, Pfkp, Aldoa, Tpi1 Gapdh, Pgk1, Pgam1, Eno1, Pkm2 and Ldha ) was decreased in the si Ad4BP/SF-1 -treated cells ( Fig. 2b ; Supplementary Fig. 2 ). Although Lhda is not formally the member of glycolytic genes, the gene is tentatively included as the member in this study. The glycolytic pathway, which converts glucose to lactate, consists of 11 reactions ( Fig. 2b ). Among them, nine reactions are potentially mediated by multiple enzymes encoded by paralogous genes ( Supplementary Fig. 2 ). Many of the paralogues are expressed in a cell preferential manner [23] , [24] . In fact, for each reaction in the series, a single gene among the paralogues was predominantly expressed in Y-1 cells, with the exception of genes encoding phosphofructokinase. For the latter case, the expression of two paralogous genes, Pfkl and Pfkp, was detected, both of which were examined in the following studies. The decreased expression of these glycolytic genes was further validated by quantitative reverse transcription–PCR (RT–PCR; Fig. 2c ); expression of steroidogenic genes was also assessed ( Supplementary Fig. 3 ). In addition to treatment with siRNA, similar results were obtained by treatment with short hairpin RNA (shRNA) targeted to Ad4BP/SF-1 , excluding the possibility that the decreased expression of the glycolytic genes was caused by off-target effects from the pooled siRNAs ( Supplementary Fig. 4 ). Downregulation of the glycolytic genes was observed in another Ad4BP/SF-1-expressing cell line, MA-10, derived from mouse testicular Leydig cells ( Supplementary Fig. 5 ), indicating that the involvement of Ad4BP/SF-1 in glycolytic gene regulation was not cell type-specific. Next, we evaluated whether the expression of genes constituting other metabolic pathways related to energy production would be affected by si Ad4BP/SF-1 treatment. Interestingly, all of the genes involved in the PPP were found to be downregulated by si Ad4BP/SF-1 treatment ( Fig. 2d ). However, the expression of genes involved in the TCA cycle and fatty acid oxidation were not coordinately affected by si Ad4BP/SF-1 treatment ( Fig. 2e ). Direct regulation of glycolytic genes by Ad4BP/SF-1 To follow up on the possibility that genes involved in glucose metabolism were regulated by Ad4BP/SF-1 in Y-1 cells, a genome-wide study using ChIP sequencing was performed to determine the binding sites of Ad4BP/SF-1. Consequently, 2,108 ChIP-peaks were identified as targets of Ad4BP/SF-1. Nucleotide motif extraction [25] , [26] from these regions revealed that an Ad4BP/SF-1 consensus binding sequence, consistent with a previously identified motif [4] , was present in more than 90% of the ChIP-peaks ( Fig. 3a ). With respect to location, 80% of the ChIP-peaks were distributed either upstream (<10 kb from the transcription start site), within (intragenic) or downstream (<10 kb from the transcription termination site; Fig. 3b ) of the target genes; this localization was enriched as compared with what would be expected if the peaks were distributed equally across the genome because the regions within 10 kb of a gene represent only 55% of the entire genome. Indeed, the enrichment was statistically significant as determined by the χ 2 test ( P <2.2 × 10 −23 ). Figure 3: Binding of Ad4BP/SF-1 to glycolytic gene loci. ( a ) The nucleotide sequence extracted from the chromatin immunoprecipitation (ChIP)-peaks of Ad4BP/SF-1 is indicated. ( b ) The ChIP-peaks were classified into four groups according to their relative positions to the nearest genes. ( c ) Genes in which the ChIP-peaks for Ad4BP/SF-1 were localized within regions ranging from 10 kb upstream to 10 kb downstream from the transcription start site were subjected to pathway analysis [27] , [28] . Term name and fold enrichment are indicated. ( d ) The ChIP-peaks are shown for the glycolytic genes, Aldoa and Eno1 . Other genes are shown in Supplementary Figs 6–9 . Blue histograms and purple bars indicate the ChIP-peaks of Ad4BP/SF-1 and H3K27Ac regions, respectively. Black boxes indicate exons. ( e ) Chromatin immunoprecipitates recovered with an anti-Ad4BP/SF-1 antibody (black) or control IgG (white) were subjected to quantitative PCR (qPCR) to detect glycolytic genes. Average values and SDs of relative amounts of the ChIP-qPCR products are shown ( e – g ). The average values of the control products were normalized to 1.0. * P <0.05, ** P <0.01, *** P <0.005. n =3. ( f ) Chromatin immunoprecipitates recovered with an anti-Ad4BP/SF-1 antibody were subjected to qPCR analysis for the glycolytic genes (black bars) and exon 7 of the Star gene, a negative control for Ad4BP/SF-1 accumulation (white bars). The average values for the Star gene locus were normalized to 1.0. * P <0.05. ** P <0.01. *** P <0.005. n =3. ( g ) ChIP-qPCR for genes involved in tricarboxylic acid cycle ( Suclg1 and Sdhb ) and steroidogenesis ( Cyp11a1 and Star ). * P <0.05, ** P <0.01. n =3. The statistical significances were examined using a two-tailed Student’s t -test ( e – g ). Full size image To evaluate which biological processes were related to the ChIP-peaks, a pathway analysis [27] , [28] was performed using the assumption that Ad4BP/SF-1 would regulate the expression of the gene nearest to a given ChIP-peak. Consistent with the results obtained from the transcriptome analysis, pathways related to energy metabolism, including glycolysis, were identified ( Fig. 3c ). Among the glycolytic genes expressed in Y-1 cells, Ad4BP/SF-1-binding sites (represented as one or two peaks) were localized in the upstream and/or intronic regions of nine genes (including the paralogues Pfkl and Pfkp ) that mediate 8 of the 11 glycolytic reactions ( Fig. 3d ; Supplementary Figs 6–9 ). The ChIP-peaks were observed <10 kb upstream of the Eno1 , Pfkl and Pkm2 genes, and within the intronic regions of the Hk1 , Pfkp , Aldoa , Gapdh , Pgam1 , Eno1 , Pkm2 and Ldha genes. Unexpectedly, no ChIP-peaks were observed in the Gpi1 , Tpi1 and Pgk1 gene loci. Nor did we observe any ChIP-peaks in the genes involved in the PPP ( Supplementary Fig. 10 ). The presence of ChIP-peaks in glycolytic gene loci as revealed by ChIP-seq was further validated using conventional ChIP assays followed by quantitative PCR (ChIP-qPCR; Fig. 3e,f ). Previous ChIP-seq [29] and ChIP-chip [30] studies revealed that estrogen-related receptor α (ERRα, NR3B1) accumulates near genes involved in the glycolytic pathway, the TCA cycle, oxidative phosphorylation and lipid metabolism; by contrast, our ChIP-seq analysis did not show any accumulation of Ad4BP/SF-1 in genes from the latter three pathways. However, as the consensus binding sequence of ERRα is shared by Ad4BP/SF-1 (refs 4 , 31 ), we used ChIP-qPCR to examine whether Ad4BP/SF-1 accumulated on the TCA cycle genes, Suclg1 and Sdhb , where ERRα accumulates. Consistent with our ChIP-seq results, the ChIP-qPCR failed to show any accumulation of Ad4BP/SF-1 on the TCA cycle genes ( Fig. 3g ). Nonetheless, it should be noted that our studies were performed with Y-1 cells cultured under conventional conditions. Ad4BP/SF-1 might accumulate near TCA cycle genes under particular culture conditions or upon physiological stimulation. Transcriptionally active regions can be characterized by particular histone modifications. Among the modifications, acetylation at H3K27 (H3K27Ac) has been established to be primarily localized to active promoter and enhancer regions [32] . Accordingly, we performed ChIP-seq for H3K27Ac [33] and examined whether the ChIP-peaks for Ad4BP/SF-1 overlapped with the H3K27Ac-containing regions. Indeed, the Ad4BP/SF-1 ChIP-peaks coincided with the H3K27Ac regions in the Aldoa , Eno1 , Hk1 , Pfkp , Gapdh and Pkm2 genes, but not in the Pfkl , Pgam1 and Ldha genes ( Fig. 3d ; Supplementary Figs 6–9 ). We next investigated whether the ChIP-peak regions for Ad4BP/SF-1 were associated with transcriptional activity using the luciferase reporter gene constructs Aldoa -Luc, Pkm2 -Luc and Eno1 -Luc ( Fig. 4a ; Supplementary Figs 11–15 ). As expected, the ChIP-peak regions exhibited transcriptional activity, and this activity was suppressed by si Ad4BP/SF-1 treatment of Y-1 cells ( Fig. 4a ). Moreover, transcription from these constructs was activated in a dose-dependent manner by ectopically expressed Ad4BP/SF-1 in HeLa and HEK293 cells, which do not express endogenous Ad4BP/SF-1 ( Fig. 4b–d ). The transcriptional activity disappeared when all putative binding sites for Ad4BP/SF-1 located in the ChIP-peak regions were mutated ( Fig. 4e–g ; Supplementary Figs 11–15 ; Table 1 ). Moreover, the direct interaction of the purified Ad4BP/SF-1 protein with the putative binding sites located in the ChIP-peak regions was demonstrated by gel mobility shift assays ( Fig. 4h–j , Supplementary Figs 11–15 , Table 2 ). Taken together, these studies strongly suggested that Ad4BP/SF-1 regulates glycolytic gene expression through these ChIP-peak regions. 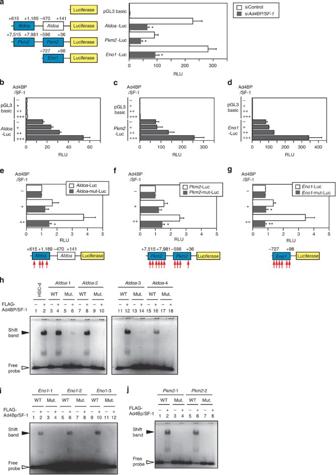Figure 4: Transactivation of glycolytic genes by Ad4BP/SF-1. (a) Luciferase reporter gene constructs, pGL3 basic,Aldoa-Luc,Pkm2-Luc andEno1-Luc, are shown. Blue squares represent genome fragments where Ad4BP/SF-1-binding was detected. A white square represents a genome fragment where Ad4BP/SF-1 binding was not detected. Numbers represent the positions of the fragments from the transcription start sites of the genes. These constructs were transfected into Y-1 cells with siAd4BP/SF-1or siControl. Average values and SDs of the luciferase activities are indicated (a–g). The average value for pGL3 basic in the siControl-treated cells was normalized to 1.0. *P<0.005.n=3. RLU; relative luciferase unit. (b–d)Aldoa–Luc (b) orPkm2–Luc (c) were transfected into HeLa cells andEno1–Luc (d) was transfected into HEK293 cells with increasing amounts of the expression vector for Ad4BP/SF-1 (ref.59). Average values for pGL3 basic in the absence of the Ad4BP/SF-1 expression vector were normalized to 1.0.n=3. +, 1 ng; ++, 5 ng; +++, 50 ng. (e–g) Luciferase reporter gene constructs,Aldoa-mut–Luc (e),Pkm2-mut–Luc (f) andEno1-mut–Luc (g), are shown at the bottom. Mutations shown inTable 1were introduced in the reporter constructs as indicated by red arrows. These mutant (Mut.) constructs (black bars) or wild-type (WT) constructs (white bars) were transfected into HeLa (e,f) or HEK293 (g) cells with increasing amounts of the expression plasmid for Ad4BP/SF-1. The average values for WT reporter genes in the absence of Ad4BP/SF-1 expression plasmid were set to 1.0. *P<0.025 (e), *P<0.05 (f), *P<0.05, **P<0.01 (g) for difference from WT reporter.n=3. +, 5 ng; ++, 50 ng. The statistical significances were examined using a two-tailed Student’st-test (a,e–g). (h–j) The oligonucleotides probes (Table 2) and purified FLAG-Ad4BP/SF-1 were used for gel mobility shift assays. A probe named Hsd-d (from humanCYP11A1gene promoter4) was used as a positive control. Direct binding of Ad4BP/SF-1 to four WT probes (Aldoa-1, 2, 3, 4) (h), three WT probes (Eno1-1, 2, 3) (i) and two WT probes (Pkm2-1, 2) (j) was observed, whereas not to the Mut probes. Figure 4: Transactivation of glycolytic genes by Ad4BP/SF-1. ( a ) Luciferase reporter gene constructs, pGL3 basic, Aldoa -Luc, Pkm2 -Luc and Eno1 -Luc, are shown. Blue squares represent genome fragments where Ad4BP/SF-1-binding was detected. A white square represents a genome fragment where Ad4BP/SF-1 binding was not detected. Numbers represent the positions of the fragments from the transcription start sites of the genes. These constructs were transfected into Y-1 cells with si Ad4BP/SF-1 or siControl. Average values and SDs of the luciferase activities are indicated ( a – g ). The average value for pGL3 basic in the siControl-treated cells was normalized to 1.0. * P <0.005. n =3. RLU; relative luciferase unit. ( b – d ) Aldoa –Luc ( b ) or Pkm2 –Luc ( c ) were transfected into HeLa cells and Eno1 –Luc ( d ) was transfected into HEK293 cells with increasing amounts of the expression vector for Ad4BP/SF-1 (ref. 59 ). Average values for pGL3 basic in the absence of the Ad4BP/SF-1 expression vector were normalized to 1.0. n =3. +, 1 ng; ++, 5 ng; +++, 50 ng. ( e – g ) Luciferase reporter gene constructs, Aldoa -mut–Luc ( e ), Pkm2 -mut–Luc ( f ) and Eno1 -mut–Luc ( g ), are shown at the bottom. Mutations shown in Table 1 were introduced in the reporter constructs as indicated by red arrows. These mutant (Mut.) constructs (black bars) or wild-type (WT) constructs (white bars) were transfected into HeLa ( e , f ) or HEK293 ( g ) cells with increasing amounts of the expression plasmid for Ad4BP/SF-1. The average values for WT reporter genes in the absence of Ad4BP/SF-1 expression plasmid were set to 1.0. * P <0.025 ( e ), * P <0.05 ( f ), * P <0.05, ** P <0.01 ( g ) for difference from WT reporter. n =3. +, 5 ng; ++, 50 ng. The statistical significances were examined using a two-tailed Student’s t -test ( a , e – g ). ( h – j ) The oligonucleotides probes ( Table 2 ) and purified FLAG-Ad4BP/SF-1 were used for gel mobility shift assays. A probe named Hsd-d (from human CYP11A1 gene promoter [4] ) was used as a positive control. Direct binding of Ad4BP/SF-1 to four WT probes ( Aldoa -1, 2, 3, 4) ( h ), three WT probes ( Eno1 -1, 2, 3) ( i ) and two WT probes ( Pkm2 -1, 2) ( j ) was observed, whereas not to the Mut probes. Full size image Table 1 Candidate sequences for Ad4BP/SF-1-binding sites ( Aldoa -1 to -4, Pkm 2-1 to -10, and Eno1 -1 to -6 as defined in Supplementary Figs 11–15 ) are mutated as shown by lower case letters. Full size table Table 2 Nucleotide sequences of the probes used in the gel mobility shift assay are listed. Full size table Glucose metabolism affected by si Ad4BP/SF-1 treatment Considering that Ad4BP/SF-1 positively regulates glycolytic and PPP gene expression, although possibly through different mechanisms, cellular glucose metabolism should be affected by si Ad4BP/SF-1 treatment. To verify this assumption, we determined the glucose concentrations in cell culture medium. Glucose concentrations decreased rapidly in medium from siControl-treated cells, but dropped slowly in medium from si Ad4BP/SF-1 -treated cells ( Fig. 5a ). Because this decrease in glucose was primarily driven by cellular uptake, and because cell numbers were decreased by si Ad4BP/SF-1 treatment, we calculated glucose uptake per cell ( Fig. 5b ). The results indicated that glucose uptake by the si Ad4BP/SF-1 -treated cells was severely decreased by comparison to the siControl-treated cells. This decreased glucose uptake could be observed with an additional siRNA, which can efficiently suppress the expression of Ad4BP/SF-1, and with MA-10 cells ( Fig. 6a,b ; Supplementary Fig. 16a,b ). Glucose uptake would be decreased by the impaired expression of glucose transporter genes mediated by si Ad4BP/SF-1 treatment. In fact, the expression of Slc2a1 , most abundantly expressed in Y-1 cells, was markedly decreased among glucose transporter and sodium/glucose cotransporter family members ( Supplementary Fig. 17 ). However, it is unlikely that Ad4BP/SF-1 directly regulates the transporter gene because ChIP-peak analysis did not reveal binding between the two analytes. 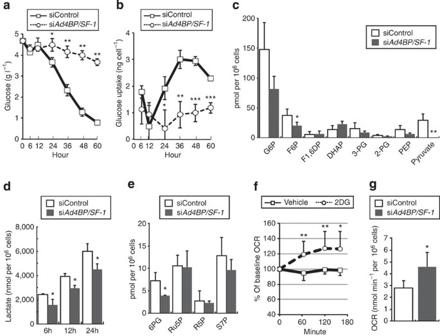Figure 5: Glucose metabolism is affected byAd4BP/SF-1knockdown in Y-1 cells. (a) Glucose concentrations were determined in culture medium from cells treated with siAd4BP/SF-1(dashed line) and siControl (solid line). Average values and SDs are indicated (a–g). *P<0.05. **P<0.005.n=3. (b) Glucose uptake per cell was calculated from the values obtained inaand is shown after normalization to the number of cells. *P<0.05. **P<0.01. ***P<0.005.n=3. (c) The amounts of glycolytic intermediates in siAd4BP/SF-1-(black bar) and siControl- (white bar) treated cells were determined by capillary electrophoresis-mass spectrometry34. *P<0.05. **P<0.005.n=4. (d) The amount of lactate in the culture media was determined at 6, 12 and 24 h after medium change (see Methods for details). *P<0.05.n=3. (e) The amount of pentose phosphate pathway intermediates in siAd4BP/SF-1-(black bar) and siControl- (white bar) treated cells was determined. *P<0.05.n=4. (f) The oxygen consumption rate (OCR) in Y-1 cells was determined at 64, 120 and 160 min after the addition of 50 mM 2-deoxyglucose (2DG) or vehicle. 2DG was used to inhibit glucose metabolism. The OCR of the cells before the addition of 2DG is set to 100%. Data are expressed as the percent change relative to the baseline rate. *P<0.05. **P<0.025.n=6. (g) The OCR was determined in Y-1 cells at 48 h after the second siAd4BP/SF-1treatment. The OCR, normalized by cell number, is indicated. *P<0.025.n=6. The statistical significances were examined using a two-tailed Student’st-test (a–g). Figure 5: Glucose metabolism is affected by Ad4BP/SF-1 knockdown in Y-1 cells. ( a ) Glucose concentrations were determined in culture medium from cells treated with si Ad4BP/SF-1 (dashed line) and siControl (solid line). Average values and SDs are indicated ( a – g ). * P <0.05. ** P <0.005. n =3. ( b ) Glucose uptake per cell was calculated from the values obtained in a and is shown after normalization to the number of cells. * P <0.05. ** P <0.01. *** P <0.005. n =3. ( c ) The amounts of glycolytic intermediates in si Ad4BP/SF-1- (black bar) and siControl- (white bar) treated cells were determined by capillary electrophoresis-mass spectrometry [34] . * P <0.05. ** P <0.005. n =4. ( d ) The amount of lactate in the culture media was determined at 6, 12 and 24 h after medium change (see Methods for details). * P <0.05. n =3. ( e ) The amount of pentose phosphate pathway intermediates in si Ad4BP/SF-1- (black bar) and siControl- (white bar) treated cells was determined. * P <0.05. n =4. ( f ) The oxygen consumption rate (OCR) in Y-1 cells was determined at 64, 120 and 160 min after the addition of 50 mM 2-deoxyglucose (2DG) or vehicle. 2DG was used to inhibit glucose metabolism. The OCR of the cells before the addition of 2DG is set to 100%. Data are expressed as the percent change relative to the baseline rate. * P <0.05. ** P <0.025. n =6. ( g ) The OCR was determined in Y-1 cells at 48 h after the second si Ad4BP/SF-1 treatment. The OCR, normalized by cell number, is indicated. * P <0.025. n =6. The statistical significances were examined using a two-tailed Student’s t -test ( a – g ). 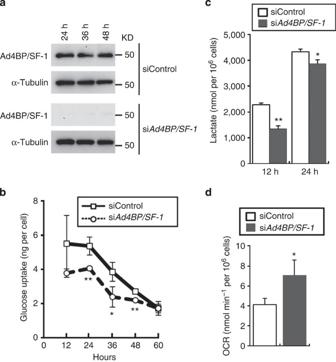Figure 6: Glucose metabolism is affected byAd4BP/SF-1knockdown in MA-10 cells. (a) Whole-cell lysates prepared from MA-10 cells treated for 24, 36 or 48 h with siControl or siAd4BP/SF-1were subjected to immunoblotting to examine the expression levels of Ad4BP/SF-1. An small interfering RNA (Mm_Nr5a1_1636, see Methods) was used. α-Tubulin was used as a control. (b) Glucose uptake per cell is indicated. Average values and SDs are shown (b–d). *P<0.05. **P<0.025.n=3. (c) The amount of lactate in the culture media was determined at 6, 12 and 24 h after medium change (see Methods for details). *P<0.025. **P<0.005.n=3. (d) The oxygen consumption rate (OCR) was determined in MA-10 cells at 48 h after the second siAd4BP/SF-1treatment. The OCR, normalized by cell number, is indicated. *P<0.01.n=6. The statistical significances were examined using a two-tailed Student’st-test (b–d). Full size image Figure 6: Glucose metabolism is affected by Ad4BP/SF-1 knockdown in MA-10 cells. ( a ) Whole-cell lysates prepared from MA-10 cells treated for 24, 36 or 48 h with siControl or si Ad4BP/SF-1 were subjected to immunoblotting to examine the expression levels of Ad4BP/SF-1. An small interfering RNA (Mm_Nr5a1_1636, see Methods) was used. α-Tubulin was used as a control. ( b ) Glucose uptake per cell is indicated. Average values and SDs are shown ( b – d ). * P <0.05. ** P <0.025. n =3. ( c ) The amount of lactate in the culture media was determined at 6, 12 and 24 h after medium change (see Methods for details). * P <0.025. ** P <0.005. n =3. ( d ) The oxygen consumption rate (OCR) was determined in MA-10 cells at 48 h after the second si Ad4BP/SF-1 treatment. The OCR, normalized by cell number, is indicated. * P <0.01. n =6. The statistical significances were examined using a two-tailed Student’s t -test ( b – d ). Full size image In addition to glucose, we also determined the levels of glycolytic intermediates by metabolomic analysis [34] ( Fig. 5c ). The levels tended to decrease following si Ad4BP/SF-1 treatment, although fructose 1,6-diphosphate (F1,6DP) and dihydroxyacetone phosphate (DHAP) levels did not decrease. Specifically, pyruvate was not detectable in the si Ad4BP/SF-1 -treated cells, presumably because the unaffected TCA cycle rapidly consumed pyruvate, whose levels were possibly decreased by the modulation in glycolytic activity. Although these results suggested that glucose metabolic activity was affected by si Ad4BP/SF-1 treatment, changes in the sizes of the glycolytic intermediate pools might not directly reflect the affected metabolic activity. Thus, we also assessed the amount of lactate in the culture medium, because lactate produced in the cytosol is excreted into the culture medium by a monocarboxylate transporter [35] . As shown in Fig. 5d , lactate levels were decreased in the culture medium from si Ad4BP/SF-1 -treated cells as compared with controls. Similar results were obtained in both Y-1 and MA-10 cells treated with the additional Ad4BP/SF-1 siRNA ( Fig. 6c ; Supplementary Fig. 16c ). In addition to the glycolytic intermediates, the amount of 6-phosphogluconate (6PG), one of the PPP intermediates ( Fig. 2b ), was significantly decreased by si Ad4BP/SF-1 treatment ( Fig. 5e ). Oxygen consumption rate (OCR) is frequently used as a proxy of cellular metabolic activity. Previous studies demonstrated that the inhibition of glycolysis leads to the activation of mitochondrial respiration, and thus, an increase in the OCR [36] , [37] . First, we examined whether this increase could be observed in Y-1 cells treated with the non-metabolizable glucose analogue, 2-deoxyglucose (2DG), which inhibits the glycolytic pathway. As expected, the OCR was increased in response to 2DG treatment ( Fig. 5f ). Because our knockdown studies strongly suggested that glucose metabolism in Y-1 cells was affected by si Ad4BP/SF-1 treatment, the OCR in the cells was assumed to be increased. Indeed, the OCR was elevated in si Ad4BP/SF-1 -treated Y-1 cells ( Fig. 5g ). A similar increase in the OCR was also observed in Y-1 and MA-10 cells treated with an additional siRNA ( Fig. 6d ; Supplementary Fig. 16d ). Decreased cell proliferation due to affected metabolism Based on changes in glucose metabolism, we hypothesized that the amount of intracellular ATP would be decreased in si Ad4BP/SF-1 -treated cells. As expected, treatment with si Ad4BP/SF-1 led to a 38% reduction in intracellular ATP ( Fig. 7a ). In order to verify that this reduction was predominantly due to effects on glucose metabolism, cells were treated with 2DG and an inhibitor for mitochondrial ATP synthase, oligomycin (OM). In siControl-treated Y-1 cells, 2DG treatment decreased ATP levels by 27% ( Fig. 7a ), whereas treatment with 2DG in combination with OM decreased ATP amounts by 85% ( Fig. 7a ), indicating that ATP production in Y-1 cells was predominantly dependent on glycolysis and oxidative phosphorylation. By contrast, in si Ad4BP/SF-1 -treated cells, ATP levels decreased only slightly by 2DG treatment ( Fig. 7a ), whereas treatment with 2DG and OM decreased ATP to levels similar to those observed in siControl-treated cells ( Fig. 7a ). Decreased ATP levels were observed in Y-1 and MA-10 cells treated with the additional Ad4BP/SF-1 siRNA ( Fig. 7b ; Supplementary Fig. 18a ). 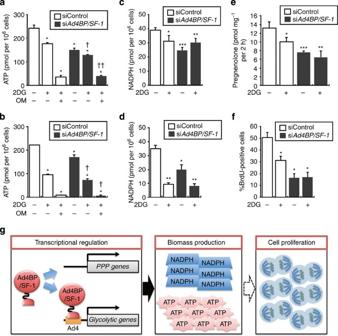Figure 7: Ad4BP/SF-1 regulates ATP/ nicotinamide adenine dinucleotide phosphate (NADPH) production and cell proliferation. (a,b) The contributions of glucose metabolism (via the glycolytic pathway) and mitochondrial oxidative phosphorylation (OXPHOS) to ATP production were examined in siAd4BP/SF-1-(black bar) and siControl- (white bar) treated Y-1 (a) and MA-10 (b) cells. 2-Deoxyglucose (2DG) and oligomycin (OM) were used to inhibit glucose metabolism and OXPHOS, respectively. Average values and SDs are shown (a–f). Bars denoted with an ‘*’ are compared with siControl-treated cells in the absence of reagents; *P<0.005 (a,b). Bars denoted with an ‘†’ are compared with siAd4BP/SF-1-treated cells in the absence of reagents;†P<0.025,††P<0.005 (a),†P<0.005 (b).n=3. (c,d) The contribution of glucose metabolism (pentose phosphate pathway (PPP)) to NADPH production was examined in siAd4BP/SF-1-(black bar) and siControl- (white bar) treated Y-1 (c) and MA-10 (d) cells.n=3. *P<0.05, **P<0.025, ***P<0.01 (c), *P<0.01, **P<0.005 (d). (e) The production of pregnenolone was examined in siAd4BP/SF-1-(black bar) and siControl- (white bar) treated Y-1 cells. *P<0.05, **P<0.025, ***P<0.01 for difference from siControl-treated cells in the absence of the reagents.n=3. (f) The effect of glucose metabolism on cell proliferation was examined in siAd4BP/SF-1-(black bar) and siControl- (white bar) treated Y-1 cells. *P<0.005.n=3. The statistical significances were examined using a two-tailed Student’st-test (a–f). (g) A proposed model based on the results of the current study. It has been established that Ad4BP/SF-1 is involved in tissue-specific gene expression. In addition to this function, the present study strongly suggests that Ad4BP/SF-1 positively regulates cell proliferation, at least in part, through the transcriptional regulation of genes responsible for the production of important coenzymes, for example, ATP and NADPH. Figure 7: Ad4BP/SF-1 regulates ATP/ nicotinamide adenine dinucleotide phosphate (NADPH) production and cell proliferation. ( a , b ) The contributions of glucose metabolism (via the glycolytic pathway) and mitochondrial oxidative phosphorylation (OXPHOS) to ATP production were examined in si Ad4BP/SF-1- (black bar) and siControl- (white bar) treated Y-1 ( a ) and MA-10 ( b ) cells. 2-Deoxyglucose (2DG) and oligomycin (OM) were used to inhibit glucose metabolism and OXPHOS, respectively. Average values and SDs are shown ( a – f ). Bars denoted with an ‘*’ are compared with siControl-treated cells in the absence of reagents; * P <0.005 ( a , b ). Bars denoted with an ‘ † ’ are compared with si Ad4BP/SF-1 -treated cells in the absence of reagents; † P <0.025, †† P <0.005 ( a ), † P <0.005 ( b ). n =3. ( c , d ) The contribution of glucose metabolism (pentose phosphate pathway (PPP)) to NADPH production was examined in si Ad4BP/SF-1- (black bar) and siControl- (white bar) treated Y-1 ( c ) and MA-10 ( d ) cells. n =3. * P <0.05, ** P <0.025, *** P <0.01 ( c ), * P <0.01, ** P <0.005 ( d ). ( e ) The production of pregnenolone was examined in si Ad4BP/SF-1- (black bar) and siControl- (white bar) treated Y-1 cells. * P <0.05, ** P <0.025, *** P <0.01 for difference from siControl-treated cells in the absence of the reagents. n =3. ( f ) The effect of glucose metabolism on cell proliferation was examined in si Ad4BP/SF-1- (black bar) and siControl- (white bar) treated Y-1 cells. * P <0.005. n =3. The statistical significances were examined using a two-tailed Student’s t -test ( a – f ). ( g ) A proposed model based on the results of the current study. It has been established that Ad4BP/SF-1 is involved in tissue-specific gene expression. In addition to this function, the present study strongly suggests that Ad4BP/SF-1 positively regulates cell proliferation, at least in part, through the transcriptional regulation of genes responsible for the production of important coenzymes, for example, ATP and NADPH. Full size image Next, we examined NADPH levels, which are produced mainly by the PPP. 2DG is metabolized to 6-phospho-2-deoxygluconate, which cannot be metabolized further in the PPP. Therefore, 2DG treatment is expected to inhibit reactions downstream of 6PG in the PPP and thus partially inhibits NADPH production in PPP ( Fig. 2b ). As expected, treatment with si Ad4BP/SF-1 reduced NADPH levels by 37% ( Fig. 7c ). Treatment of control cells with 2DG also reduced NADPH production, but to a lesser extent than si Ad4BP/SF-1 treatment ( Fig. 7c ). This modest decrease in NADPH by 2DG treatment might be attributable to the fact that 1 mol of NADPH is produced in the reaction from 2DG to 6-phospho-2-deoxygluconate ( Fig. 2b ). Although the reasons are unclear, NADPH levels in si Ad4BP/SF-1 -treated cells were slightly restored by 2DG treatment. Treatment with the additional Ad4BP/SF-1 siRNA decreased NADPH levels in Y-1 and MA-10 cells ( Fig. 7d ; Supplementary Fig. 18b ). Together, the decrease in both NADPH and steroidogenic gene expression mediated by siRNAs ( Supplementary Fig. 3 ) suggested that steroid production would be affected in Y-1 cells. In fact, pregnenolone production under adrenocorticotropic hormone stimulation was decreased by si Ad4BP/SF-1 treatment, possibly due to the changes in both NADPH production and steroidogenic gene expression levels ( Fig. 7e ). Finally, we examined the relationship between glucose metabolism and cell proliferation. Treatment of control cells by 2DG decreased cell proliferation by 38% ( Fig. 7f ), whereas treatment with si Ad4BP/SF-1 had an even greater impact on cell proliferation ( Fig. 7f ), which was not further affected by co-treatment with 2DG ( Fig. 7f ). Similar results were obtained by counting cell numbers ( Supplementary Fig. 19 ). Taken together, the data suggested the possibility that Ad4BP/SF-1 regulates cell proliferation, at least in part, by mediating the transcriptional regulation of the genes responsible for the production of vital coenzymes, for example, ATP and NADPH ( Fig. 7g ). Our transcriptomic and metabolomic analyses, together with ChIP-seq experiments, revealed that Ad4BP/SF-1 is involved in glucose metabolism by regulating genes for the glycolytic pathway and PPP, both of which are pivotal housekeeping processes. Glucose is catabolized in the glycolytic pathway to produce ATP, whereas it is catabolized in the PPP to produce NADPH and ribose. All of these products are essential for cellular function and for the generation of daughter cells [38] , [39] . Considering our finding that Ad4BP/SF-1 regulates glucose metabolism, it seems plausible that disruption of the Ad4BP/SF-1 gene in vivo could lead to an insufficient production of ATP and NADPH through impaired activation of glucose metabolism, and thereby result in dysgenesis of steroidogenic tissues. It is interesting to note that Ad4BP/SF-1 is probably involved in the regulation of housekeeping genes required for glucose metabolism, even though it has previously been established as a tissue-specific transcription factor regulating all steroidogenic gene expression in the gonads and adrenal cortex. Cholesterol is the raw material used for steroid hormone synthesis, and it is supplied to steroidogenic cells through two main supply routes: (1) incorporation from the blood and (2) de novo synthesis from acetyl-CoA through multiple enzymatic steps [40] , [41] . In fact, testicular Leydig cells synthesize a certain percentage of their intracellular cholesterol supplies [42] . Notably, both ATP and NADPH are consumed in the cholesterol synthetic pathway. In addition, NADPH is also required for P450-mediated reactions in the steroid hormone synthetic pathway [43] . Considering the requirement for ATP and NADPH in de novo steroidogenesis from acetyl-CoA, it seems likely that the genes involved in glucose metabolism could be activated cooperatively in steroidogenic cells with the genes involved in steroidogenesis. Moreover, this cooperative regulation of biomass supply and demand for steroidogenesis would be possible if a single key transcription factor were implicated in both pathways. Our results show that Ad4BP/SF-1 is a plausible candidate to orchestrate tissue-specific steroidogenic gene regulation and housekeeping glucose metabolic gene regulation, thereby enabling tissue-specific functions. As Ad4BP/SF-1 -deficient mice die shortly after birth with dysgenesis of the adrenal gland and gonads, evaluating the postnatal effects of the gene under null conditions was a challenge. To overcome this limitation, pituitary gonadotrope- and gonad-specific Ad4BP/SF-1- deficient mice were generated [44] , [45] . As expected, these mice survived postnatally, although they displayed structurally and functionally impaired tissues. Although these studies revealed crucial roles for Ad4BP/SF-1 in tissue development, the involvement of Ad4BP/SF-1 in the regulation of glucose metabolism remains to be investigated. The ventromedial hypothalamic (VMH) nucleus is known to regulate energy homeostasis through the control of food intake and energy expenditure. The production of VMH-specific Ad4BP/SF-1 -deficient mice that could survive postnatally allowed for experiments that linked the loss of Ad4BP/SF-1 with high-fat diet-induced obesity and impaired thermogenesis [46] . Although the precise mechanisms underlying these connections remain to be delineated, it might be noteworthy that the expression of genes participating in metabolic regulation, for example, the leptin receptor, was downregulated in VMH-specific Ad4BP/SF-1 null animals. Although we do not yet know whether Ad4BP/SF-1 regulates glycolytic genes in the VMH, it is noteworthy that the leptin receptor may be directly regulated by Ad4BP/SF-1 (ref. 47 ). Together, these data suggest that Ad4BP/SF-1 coordinates whole body glucose metabolism by enabling the VMH to sense energy states. The tissue-specific expression of Ad4BP/SF-1 raises the question as to which transcription factor regulates glucose metabolism in other cell types. In this regard, it is interesting to note the function of the ERRα (NR3B1). As Ad4BP/SF-1 and ERRα bind to essentially same nucleotide sequence in order to exert their transcriptional activities [4] , [31] , it is likely that both factors share target genes. A ChIP-Chip analysis [30] and a recent ChIP-seq study of mouse liver [29] demonstrated that ERRα is involved in the regulation of genes involved in energy metabolism, including glycolysis, the TCA cycle, oxidative phosphorylation and lipid metabolism. Moreover, Drosophila ERR was also shown to regulate glycolytic gene expression in mid-embryogenesis [46] . Accordingly, with a focus on glycolytic genes, we compared the ChIP-seq data sets for Ad4BP/SF-1 and ERRα. As shown in Supplementary Fig. 20 , the ChIP-peaks for Ad4BP/SF-1 and ERRα clearly overlapped for seven glycolytic gene loci, whereas ChIP-peaks for each effector, albeit not overlapped, were detected for three other genes. Therefore, the two nuclear receptors seem to regulate most glycolytic genes by binding to the same genetic loci. However, considering that Ad4BP/SF-1 is expressed only in endocrine tissues, for example, the adrenal cortex and gonads [3] , [10] , whereas ERRα is expressed in a broad range of tissues [48] , the contribution of these two nuclear receptors to glycolytic gene regulation likely varies among tissues. The differences in the materials for this ChIP-seq study as compared with the previous one notwithstanding, it is interesting to note that Ad4BP/SF-1 did not accumulate in genes involved in the TCA cycle or oxidative phosphorylation. There may be a few possible explanations for the apparent differential accumulation of effectors between the two studies. First, the nucleotide sequences surrounding the binding sites may affect the binding of Ad4BP/SF-1 and ERRα. Second, the physiological condition of the Y-1 cells and the mouse liver used for the two studies might be different. Under disparate conditions, the two nuclear receptors may work differentially. Finally, as Y-1 cells were derived from adrenocortical tumor cells, the glycolytic pathway may be accelerated in those cells, as in other tumor cells [49] . Thus, the impact of Ad4BP/SF-1 on glycolytic gene regulation might be accentuated in Y-1 cells. An investigation of these possibilities would help to delineate the mechanisms underlying the selection of differential target genes between Ad4BP/SF-1 and ERRα. A group of genes that control related functions and are regulated together by an inducer or repressor has been defined as a regulon [50] . Although the binding of Ad4BP/SF-1 is not observed in all glycolytic gene loci and thus the term ‘regulon’ does not formally apply in this case, the results obtained by the knockdown study and ChIP-seq suggest the possibility that glycolytic genes are regulated as an Ad4BP/SF-1 regulon in Y-1 cells. Therefore, our study with Ad4BP/SF-1, together with the ERRα study, raises the possibility that a subset of closely related nuclear receptors governs glucose metabolism. In addition, considering that the nucleotide sequence recognized by Ad4BP/SF-1 can be shared by NR5A2 (LRH1) [51] , and at least in part by NR4 family members [52] , [53] , these nuclear receptors may share target genes. Although Charest-Marcotte et al. referred to the set of genes regulated by ERRα as an ‘ERRα regulon’ [30] , our study provides the possibility that a subset of nuclear receptors may regulate metabolic processes through constructing regulons. Moreover, our present study provides, for the first time, the possibility that a single nuclear receptor governs cellular growth/maintenance and tissue-specific functions by balancing biomass supply and demand. Knockdown of Ad4BP/SF-1 Y-1 cells were transfected with a mixture of three siRNA duplexes (stealth RNAi; Nr5a1-MSS240944: 5′-UUAAAGACCAUGCACCUUCGUGCCC-3′, Nr5a1-MSS240945: 5′-ACAAGGUGUAAUCCAACAGGGCAGC-3′ and Nr5a1-MSS240946: 5′-AAUAGCAACUGCUGGAAUUUGUCCC-3′, Invitrogen) using the Lipofectamine RNAiMAX reagent (Invitrogen) according to the manufacturer’s instructions for 48 h. When siRNA treatment continued for more than 48 h, the cells were detached once from the dish at 48 h after the first transfection, and re-seeded with the RNAiMAX reagent containing the siRNA mixture. The cells were harvested at the indicated time points. A control siRNA (Stealth RNAi Negative Control Medium GC Duplex, Invitrogen) was used as a negative control. To rule out potential off-target effects of the siRNA mixture used, we performed knockdown of Ad4BP/SF-1 by another siRNA (Mission siRNA; Mm_Nr5a1_1636: 5′-CAUUACACGUGCACCGAGATT-3′, Sigma; Figs 6 and 7b,d,e , Supplementary Figs 5, 16 and 18 ) and shRNA (shsf1#3: 5′-CGUCUGUCUCAAGUUCCUCAU-3′; Supplementary Fig. 4 ). For negative control of shRNA experiment, shluc: 5′-CCUAAGGUUAAGUCGCCCUCG-3′ was used. RT–PCR Total RNA was prepared from Y-1 cells treated with si Ad4BP/SF-1 or siControl. cDNA was synthesized from the RNA using M-MLV reverse transcriptase (Invitrogen), and then subjected to quantitative RT–PCR. Real-time PCR was performed with an ABI 7500 real-time PCR system (Applied Biosystems) using THUNDERBIRD SYBR qPCR mix (Toyobo). Primers used for RT–PCR are listed in the Supplementary Table 2 . Immunoblot Whole-cell extracts were prepared from Y-1 cells treated with si Ad4BP/SF-1 or siControl using lysis buffer (50 mM Tris–HCl pH 8.0, 50 mM NaCl, 1 mM EDTA and 1% SDS). After the protein concentration was determined using a BCA Protein Assay Kit (Pierce Biotechnology), 10 μg of whole-cell extract was subjected to SDS–polyacrylamide gel electrophoresis, followed by immunoblotting. Anti-Ad4BP/SF-1 antiserum (1:1,000) or an anti-α−tubulin antibody (T-9026, Sigma-Aldrich 1:1,000) was used as the primary antibodies. Anti-rabbit donkey IgG (1:1,000) and anti-mouse donkey IgG (GE Healthcare, 1:1,000) were used as secondary antibodies. Bound antibodies were detected using an ECL Plus Western Blotting Detection System (GE Healthcare). mRNA-seq Poly-A+ RNA was prepared from si Ad4BP/SF-1 or siControl-treated Y-1 cells using oligo(dT) magnetic beads. The library for mRNA-seq was prepared using the TruSeq RNA Sample Prep Kit v2 (Illumina) according to the manufacturer’s instructions. After the quality of the library was validated using the Agilent Bioanalyzer 2100 (Agilent Technologies), the samples were subjected to sequencing with a next-generation sequencer (GAIIx, Illumina). Mapping and quantification of gene expression were performed by Tophat [54] and Cufflinks [55] . mRNA-seq data processing The RNA-seq reads were aligned to the reference mouse genome sequence, UCSC mm9 (NCBI 37) using the TopHat [54] programme version 1.4.1 with the default parameters. Cufflinks [55] (version 1.3.0) was then used to assemble the transcripts and to calculate fragments per kilobase of transcript per million mapped fragments with the default parameters. ChIP-qPCR and ChIP-seq ChIP assays were performed according to the procedure described by Winnay and coworkers [56] . Briefly, Y-1 cells were fixed with 1% formaldehyde for 5 min at room temperature, and then glycine was added to a final concentration of 125 mM to stop the crosslinking reaction. Then, the fixed cells were lysed with ChIP lysis buffer (50 mM Tris–HCl pH 8.0, 10 mM EDTA, 1% SDS), followed by sonication (UCD-300 Bioruptor, Diagenode, Belgium). After diluting the SDS by adding nine volumes of dilution buffer (20 mM Tris–HCl pH 8.0, 2 mM EDTA, 150 mM NaCl, 1% Triton X-100), the sheared chromatin was subjected to immunoprecipitation with anti-Ad4BP/SF-1 or anti-H3K27Ac antibodies. The immunoprecipitates were collected using Dynabeads with Protein A (Life Technologies), and were sequentially washed with ChIP-RIPA buffer (50 mM Tris–HCl pH 8.0, 5 mM EDTA, 150 mM NaCl, 0.1% SDS, 0.5% NP-40), high-salt ChIP-RIPA buffer (50 mM Tris–HCl pH 8.0, 5 mM EDTA, 500 mM NaCl, 0.1% SDS, 0.5% NP-40), LiCl buffer (10 mM Tris–HCl pH 8.0, 1 mM EDTA, 250 mM LiCl, 0.1% NP-40) and TE buffer (10 mM Tris–HCl pH 8.0, 1 mM EDTA). Finally, the chromatin fragments were eluted from the beads with elution buffer (0.1 M NaHCO 3 , 1% SDS, 10 mM dithiothreitol). After the crosslinks were reverted by heating at 65 °C for 16 h, DNA fragments were purified using the QIAquick PCR Purification kit (Qiagen). For ChIP-qPCR, the purified DNAs were subjected to real-time PCR using primer sets listed in Supplementary Table 2 . For ChIP-seq, the DNA fragments were used to prepare the ChIP-seq library with NEBNext DNA sample prep master mix set 1 (New England BioLabs) and DNA sample prep kit, oligo only (Illumina) according to the manufacturer’s instructions. During the library preparation, 200 and 500 bp adaptor-ligated DNA fragments were recovered and used for the following steps. After the quality of the library was validated using the Agilent Bioanalyzer 2100 (Agilent Technology), the ChIP-seq library was subjected to sequencing with a next-generation sequencer (GAIIx, Illumina). Mapping of the sequence data was performed by Bowtie [57] . Thereafter, the mapping data were subjected to peak-calling using MACS (Model-based Analysis for ChIP-Seq) [58] . ChIP-seq data processing ChIP-seq reads were mapped to the reference mouse genome (mm9/NCBI 37) using the Bowtie [57] programme version 0.12.7, allowing up to three mismatches. The multiple-hit reads were excluded, and only the uniquely mapped reads to the reference mouse genome were kept for further analysis. To identify peaks and regions of Ad4BP/SF-1 and H3K27Ac enrichment, the uniquely mapped reads were analysed using the MACS [58] programme version 1.4.2 with the option ‘—nomodel’. The threshold P -values for enriched regions of Ad4BP/SF-1 and H3K27Ac were set to 10 −3 and 10 −5 , respectively. We prepared ChIP-seq library from DNA isolated from soluble chromatin used for chromatin immunoprecipitation, and read the sequence as input reads. The input reads were used to normalize the background noise. For 2,108 Ad4BP/SF-1 peak regions revealed by MACS, we conducted further analysis with the motif extraction programme, Discriminative Regular Expression Motif Elicitation [25] , in the Multiple Em for Motif Extraction Suite [26] , with the E -value threshold of 0.05. Average length of sequences used for the analysis is 1,388.9 bp. The option ‘-maxk’, which specifies the maximum width of the motif core, was set to nine according to the previously identified Ad4BP/SF-1 consensus motif [4] . The background sequences for DNA motif detection were generated from a set of DNA sequences with the same nucleotide composition to the peak regions. For pathway analysis, we used the MSigDB (Molecular Signature Database) [28] pathway analysis version 1.8 on the Genomic Regions Enrichmemt of Annotations Tool [27] web site ( http://bejerano.stanford.edu/great/public/html/index.php ). In this analysis, we set a rule that the single nearest gene located within 10 kb from each ChIP peak is the associated gene and the genes identified were subjected to the analysis. Luciferase reporter assay Y-1 cells were grown in DMEM (Wako) supplemented with 10% fetal bovine serum and 1 × penicillin-streptomycin (Invitrogen) on 24-well plates (Iwaki, Tokyo, Japan). pGL3-basic (Promega Corp.), Aldoa -Luc, Pkm2 -Luc and Eno1 -Luc ( Supplementary Figs 11–15 ) were transfected with si Ad4BP/SF-1 or siControl into Y-1 cells using the Lipofectamine 2000 transfection reagent (Invitrogen). Human cervical adenocarcinoma-derived HeLa and human embryonic kidney-derived HEK293 cells were grown in DMEM (Wako) supplemented with 10% fetal bovine serum and 1 × penicillin-streptomycin on 24-well plates (Iwaki). The wild-type or mutant luciferase reporters ( Table 1 ) were transfected with increasing amounts of Ad4BP/SF-1 expression plasmid [59] into HeLa or HEK293 cells. pCMV-SPORT-βgal (Invitrogen) was used as an internal control. Six hours after transfection, the medium was replaced. Forty-eight hours after transfection, the cells were harvested, and luciferase and β-galactosidase activities were determined. Gel mobility shift assay Purified Ad4BP/SF-1 protein was prepared as described [60] and the protein was incubated with the oligonucleotide probes (sequences are listed in Table 2 ) in a binding buffer (15 mM HEPES-KOH (pH 7.9), 1 mM EDTA, 4% Ficoll and 250 mM KCl) for 30 min at 4 °C. Then, the reaction products were subjected to polyacrylamide gel electrophoresis. The gel was stained with SYBR Gold nucleic acid gel stain for 30 min (Invitrogen). Measurements of glucose and lactate levels Six hours after the second siRNA treatment (see siRNA treatment method for details), the medium was replaced. At 6, 12, 24, 36, 48 and 60 h after the medium exchange, small volumes of the culture media were sampled. Glucose and lactate concentrations in the conditioned media were measured using the Glucose (HK) Assay Kit (Sigma) and the Lactate Assay Kit (BioVision Inc.), respectively, according to the manufacturers’ instructions. Measurement of OCR The OCR of Y-1 cells was measured using an XF24 extracellular Flux Analyzer (Seqhorse Bioscience), according to the manufacturer’s instructions. Forty-eight hours after the second siRNA treatment, Y-1 cells were subjected to analysis. Measurement of ATP levels Measurement of ATP levels was performed according to the procedure described by Yagi and co-workers [61] . Forty-eight hours after the second siRNA treatment, Y-1 cells were treated with 20 mM 2DG (Nacalai Tesque, Inc.) for 4 h, followed by a 30-min incubation with 10 μM OM (Cell Signaling Technology, Inc). The cells were lysed in the lysis buffer (Promega), and cellular ATP levels were measured using an ATP-determination kit (Promega) according to the manufacturer’s instructions. Measurement of NADPH levels Forty-eight hours after the second siRNA treatment, Y-1 cells were treated with 20 mM of 2DG for 4 h, and then the cells were harvested. Cellular NADPH levels were measured using a NADP+/NADPH Quantification Kit (BioVision Inc.) according to the manufacturer’s instruction. Measurement of pregnenolone production Forty-eight hours after transfection of siControl or si Ad4BP/SF-1 (Mission, siRNA, Mm_Nr5a1_1636), 2-3 × 10 6 Y-1 cells were incubated with 2 ml DMEM containing 1 nM adrenocorticotropic hormone (Cortrosyn, Daiichi Sankyo CO., LTD). 2 μM trilostane (kindly supplied by Dr Mizuno, Mochida Pharmaceutical CO., LTD) was also added to inhibit 3β-hydroxysteroid dehydrogenase (Hsd3b1), which mediates conversion from pregnenolone to progesterone. After incubation for 2 h with or without 20 mM 2DG, the medium were collected and subjected to measurement of pregnenolone by radioimmuno assays as described previously [62] , [63] . The amount of pregnenolone was normalized with total amount of cellular protein. Cell proliferation analysis Cell proliferation was examined by 5-bromodeoxyuridine (BrdU) incorporation in si Ad4BP/SF-1- and siControl-treated cells. The siRNA-treated cells were cultured with 100 μM BrdU (Sigma) for 1.5 h after a 4-h incubation in the presence of 2DG. After fixation with paraformaldehyde, immunohistochemical analysis was performed with antibodies against BrdU (Roche). The number of BrdU-immunoreactive cells was counted to evaluate cell proliferation. Quantification of intermediates in the glycolytic pathway Forty-eight hours after the second transfection of si Ad4BP/SF-1 or siControl, extracts were prepared from more than 6.0 × 10 6 cells with methanol containing an internal standard solution (Human Metabolome Technologies). The amount of intermediate metabolites was determined using capillary electrophoresis in line with an electrospray ionization time-of-flight mass spectrometry (ESI-TOF/MS) system [34] . Statistical analysis All experiments were performed in at least three independent experimental replicates. Data are presented as the mean and standard deviation. In most instances the statistical significance was examined using a two-tailed Student’s t -test; however, for the ChIP-peak localization studies, significance was determined using the χ 2 test. Accession codes: ChIP-seq and mRNA-seq data have been deposited in DDBJ/EMBL/GenBank DRA000853. How to cite this article: Baba, T. et al. Glycolytic genes are targets of the nuclear receptor Ad4BP/SF-1. Nat. Commun. 5:3634 doi: 10.1038/ncomms4634 (2014).